High quality-factor optical nanocavities in bulk single-crystal diamond Single-crystal diamond, with its unique optical, mechanical and thermal properties, has emerged as a promising material with applications in classical and quantum optics. However, the lack of heteroepitaxial growth and scalable fabrication techniques remains the major limiting factors preventing more wide-spread development and application of diamond photonics. In this work, we overcome this difficulty by adapting angled-etching techniques, previously developed for realization of diamond nanomechanical resonators, to fabricate racetrack resonators and photonic crystal cavities in bulk single-crystal diamond. Our devices feature large optical quality factors, in excess of 10 5 , and operate over a wide wavelength range, spanning visible and telecom. These newly developed high-Q diamond optical nanocavities open the door for a wealth of applications, ranging from nonlinear optics and chemical sensing, to quantum information processing and cavity optomechanics. All contemporary integrated nanophotonic platforms have one important feature in common: they consist of a device layer—an optically thin film—supported by a substrate of a different material. The substrate provides optical isolation either by having a smaller refractive index than the device layer, or by its selective removal [1] . Single-crystal diamond is one example from an extensive list of materials—many with attractive optical properties—for which high-quality thin film heterolayer structures do not exist. Despite wafer-scale polycrystalline diamond thin films on foreign substrates being readily available, these films typically exhibit inferior properties due to scattering and absorption losses at grain boundaries, significant surface roughness and large interfacial stresses [2] , [3] , [4] . In the absence of suitable heteroepitaxial diamond growth, substantial efforts by the diamond photonics and quantum optics community have focused on novel processing techniques to yield nanoscale single-crystal diamond optical elements [5] , [6] , [7] , [8] , [9] , [10] , [11] . For the most part, these efforts have involved heterogeneous integration of single-crystal diamond slabs (~5- to 30-μm thick) on supporting silica substrates, with subsequent oxygen plasma etching to thin the slab near a target thickness ~500-nm or less. Ring resonators [12] , [13] , [14] , [15] and photonic crystal cavities [16] , [17] have been realized in such thinned diamond membranes, with recent results [18] demonstrating ultrahigh-quality factors (Q) in excess of 10 6 . While this approach remains promising [19] , complications due to material handling, scalability, repeatability and sheer difficulty of removing tens of microns of diamond while preserving uniform hundred-nanometre scale films limit this approach significantly. In this work we demonstrate state-of-the art nanophotonic resonators in single-crystal diamond substrates, realized by angled-etching [20] : an unconventional, yet scalable fabrication technique. Specifically, we realize suspended racetrack resonators and nanobeam photonic crystal cavities fabricated from a starting bulk diamond substrate. Our devices feature large optical quality factors, in excess of 10 5 , and operate over a wide wavelength range, spanning visible and telecom. These newly developed high-Q diamond optical nanocavities open the door for a wealth of applications, ranging from nonlinear optics and chemical sensing, to quantum information processing and cavity optomechanics. Angled-etching nanofabrication Our angled-etching approach, depicted in Fig. 1a–e with details summarized in Methods, employs anisotropic oxygen-based plasma etching at an oblique angle to the substrate surface, resulting in suspended structures with triangular cross-section. Angled-etching is performed in a standard inductively coupled plasma-reactive ion etcher (ICP-RIE); however, the diamond substrate is housed within a specifically designed aluminium Faraday cage that modifies the trajectory of the incident plasma ions towards the sample surface (refer to Supplementary Methods subsection (i) and Supplementary Fig. 1 for additional description of the angled-etching technique and Faraday cage designs). Importantly, diamond resonators fabricated in this way, shown in Fig. 1f,g , feature optical Q-factors on par with those found in devices realized in standard materials (for example, silicon), using conventional (planar) microfabrication techniques. 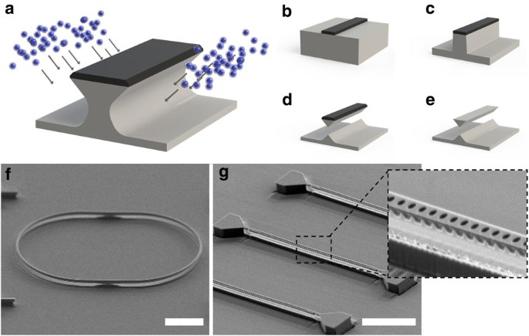Figure 1: Angled-etching fabrication methodology. (a) Illustration of angled-etching used to realize free-standing structures in bulk single-crystal diamond. (b–e) Angled-etching fabrication steps: (b) define an etch mask on substrate via standard fabrication techniques, (c) transfer etch mask pattern into the substrate by conventional top down plasma etching, (d) employ angled-etching to realize suspended nanobeam structures, (e) remove residual etch mask. Scanning electron microscope (SEM) images of (f) a fabricated diamond racetrack resonator supported from the bottom and (g) a fabricated diamond nanobeam photonic crystal cavity operating at visible wavelengths. Scale bars for SEM images inf,gcorrespond to 10 and 5 μm, respectively. All SEM images were taken at a 60° stage tilt. Figure 1: Angled-etching fabrication methodology. ( a ) Illustration of angled-etching used to realize free-standing structures in bulk single-crystal diamond. ( b – e ) Angled-etching fabrication steps: ( b ) define an etch mask on substrate via standard fabrication techniques, ( c ) transfer etch mask pattern into the substrate by conventional top down plasma etching, ( d ) employ angled-etching to realize suspended nanobeam structures, ( e ) remove residual etch mask. Scanning electron microscope (SEM) images of ( f ) a fabricated diamond racetrack resonator supported from the bottom and ( g ) a fabricated diamond nanobeam photonic crystal cavity operating at visible wavelengths. Scale bars for SEM images in f , g correspond to 10 and 5 μm, respectively. All SEM images were taken at a 60° stage tilt. Full size image Diamond racetrack resonators operating at telecom wavelengths Of the myriad of on-chip optical cavities demonstrated to date, ring and racetrack resonators are arguably the most ubiquitous [21] . Conceptually, the optical cavity is a waveguide looped back on itself, and the resonance is formed when the optical path length is an integer multiple of the wavelength. In the context of angled-etching, creating a free-standing looped waveguide represents a challenge, since suspended devices must be supported by at least one physical attachment to the bulk substrate. While free-standing wheel-and-spoke optical cavity structures [20] , [22] , [23] are an intuitively obvious solution, spoke attachment points to the looped triangular cross-section waveguide are difficult to fabricate, resulting in significant scattering losses. To circumvent this, we have developed novel vertical support structures, shown in Fig. 2a–c , and used it to realize single-crystal diamond racetrack resonators. This was accomplished by positively tapering the width of the 20-μm-long straight portions of the racetrack resonator by 15% of the nominal value. Note, an ~50° etch angle (designated as the semi angle at the bottom apex of the triangular cross-section) was used to fabricate diamond racetrack resonators shown in Fig. 2 . Refer to Supplementary Fig. 2 and Supplementary Discussion subsection (i) for cross-sectional analysis of fabrication diamond nanobeams. In angled-etching [20] , wider features require more time to be fully released from the substrate, since the structure thickness ( t ) is intrinsically linked to its width ( w ) by the etch angle ( θ ), via the relationship t = w /(2 tan θ ). As a consequence, wider sections can remain attached to the substrate resulting in a pedestal-like support at their centre. At the same time, the tapered nature of the vertical support structure minimizes optical losses (see Supplementary Fig. 3 and Supplementary Discussion subsection (ii) for modal analysis of vertically supported diamond waveguides). 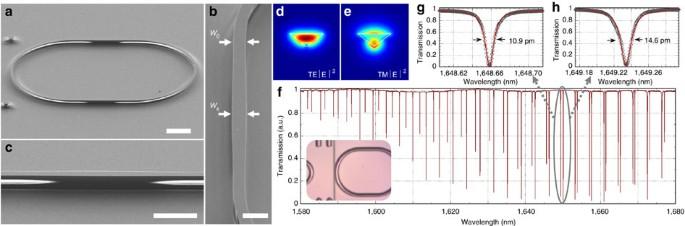Figure 2: High-Q diamond racetrack resonators. SEM images of (a) 25-μm-bend radius diamond racetrack resonator, with close-up (b) side and (c) top views. The nominal (wo) and maximum (ws) width (indicated on figure) of the tapered vertical are ~1.1 and 1.27 μm, respectively. Note, an ~50° etch angle was used to fabricate devices shown. Scale bars for SEM images ina–ccorrespond to 10, 5 and 2 μm, respectively. All SEM images were taken at a 60° stage tilt. Simulated quasi- (d) TE-like and (e) TM-like mode profiles (λ=1.55 μm, electric field norm) of a suspended 1.1-μm-wide diamond waveguide. (f) Representative normalized broadband spectrum of a 1.1-μm-wide and 37.5-μm-bend radius diamond racetrack resonator collected by fibre taper measurement. Inset shows optical micrograph indicating the fibre taper coupling position. High-resolution spectra of near critically coupled (g) TE-like and (h) TM-like modes, with Lorentzian fits to the data also shown. Lorentzian fits ing,hyield loaded Q-factors ofQL,TE~151,000 andQL,TM~113,000, respectively. Figure 2: High-Q diamond racetrack resonators. SEM images of ( a ) 25-μm-bend radius diamond racetrack resonator, with close-up ( b ) side and ( c ) top views. The nominal ( w o ) and maximum ( w s ) width (indicated on figure) of the tapered vertical are ~1.1 and 1.27 μm, respectively. Note, an ~50° etch angle was used to fabricate devices shown. Scale bars for SEM images in a – c correspond to 10, 5 and 2 μm, respectively. All SEM images were taken at a 60° stage tilt. Simulated quasi- ( d ) TE-like and ( e ) TM-like mode profiles ( λ =1.55 μm, electric field norm) of a suspended 1.1-μm-wide diamond waveguide. ( f ) Representative normalized broadband spectrum of a 1.1-μm-wide and 37.5-μm-bend radius diamond racetrack resonator collected by fibre taper measurement. Inset shows optical micrograph indicating the fibre taper coupling position. High-resolution spectra of near critically coupled ( g ) TE-like and ( h ) TM-like modes, with Lorentzian fits to the data also shown. Lorentzian fits in g , h yield loaded Q-factors of Q L,TE ~151,000 and Q L,TM ~113,000, respectively. Full size image A typical normalized transmission spectrum collected by tunable laser and photodiode from diamond racetrack resonator is shown in Fig. 2f . Fibre taper coupling [24] was used in the characterization of these devices (see Methods). Two distinct sets of transmission dips are observed, corresponding to fundamental quasi-transverse electric (TE-like) and transverse magnetic (TM-like) modes of the structure, shown Fig. 2d,e , respectively. Nearly critically coupled resonances displayed in Fig. 2g,h reveal loaded Q-factors of Q L,TE ~151,000 and Q L,TM ~113,000, where the subscript indicates the cavity mode transverse polarization. We note that the term loaded Q-factor refers to the Q-factor that includes losses due to fibre taper coupling, and at critical coupling is half the intrinsic Q-factor (that is, Q L =½ Q i ). The latter is determined by losses due to scattering, material absorption, leakage to the substrate (if any) and waveguide bends/overlaps. From our measurements, we estimate intrinsic Q-factors to be Q i,TE ~302,000 and Q i,TM ~226,000. From measured Q-factors, an upper limit on the diamond waveguide transmission loss ( α ) is estimated to be ~1.5 dB cm −1 for both guided modes via the relationship [25] : , where n g is the mode group index and λ is the resonant wavelength. While this loss value is roughly five times greater than that recently reported for single-crystal diamond waveguides fabricated via the membrane-thinning approach [18] , it is also an order of magnitude smaller than losses of polycrystalline diamond ring resonators [26] . Diamond nanobeam cavities operating at telecom wavelengths We have also fabricated diamond photonic crystal nanobeam cavities [27] using our angled-etching approach. These devices consist of a waveguide perforated with a chirped lattice of elliptically shaped air holes, which has been engineered to support resonances with ultrahigh Q -factors and ultra small mode volumes [28] . 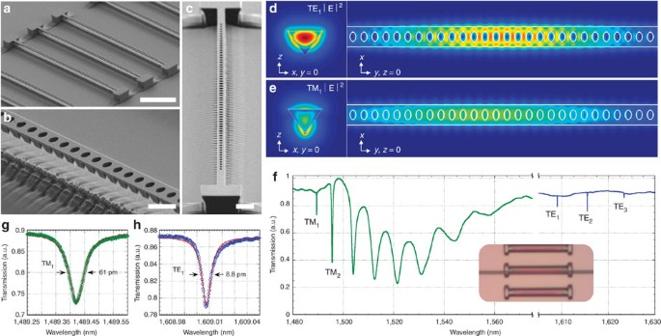Figure 3: High-Q diamond nanobeam photonic crystal cavities. SEM images of (a) diamond nanobeam photonic crystal cavities, with close-up (b) prospective and (c) top down views. Note, an ~35° etch angle was used to fabricate devices shown. Scale bars for SEM images ina–ccorrespond to 10, 1 and 2 μm, respectively. All SEM images were taken at a 60° stage tilt. Simulated cross-sectional and top down electric field intensity profiles of the fundamental quasi- (d) TE-like and (e) TM-like nanobeam photonic crystal cavity modes. Note, top down mode profiles correspond to top face of the nanobeam cavity. Theoretical figures of merit for the fundamental nanobeam photonic crystal cavity modes are Q-factors ofQTM~1.3 × 105andQTE~3.0 × 106, with mode volumesVTM~2.55(λ/n)3andVTE~2.26(λ/n)3(the subscript refers to the cavity mode transverse polarization). (f) Representative normalized broadband spectrum of a fabricated diamond photonic crystal cavity collected by fibre taper measurement, with inset optical micrograph indicating the fibre taper coupling position. High-resolution spectra of the fundamental (g) TM-like and (h) TE-like cavity modes, with Lorentzian fits to the data also shown. The taper-loaded Q-factors (extracted from Lorentzian fits to the data) of the fundamental and second-order TM-like cavity modes were 24,000 and 3,700, respectively, while the first three TE-like cavity modes had loaded Q-factors of 183,000, 94,000 and 22,000, respectively. Figure 3a–c displays a representative single-crystal diamond nanobeam cavity fabricated with etch angle θ ~35° for operation in the telecom band (see Supplementary Fig. 2 and Supplementary Discussion subsection (i) for cross-sectional analysis of fabrication diamond nanobeams). Since the nanobeam thickness and width are linked through angled-etching, global scaling of the nanobeam cavity dimensions results in tuning of the cavity resonance while maintaining all cavity figures of merit (that is, Q-factor and mode volume). Therefore, the nanobeam cavity design used in this work is parameterized by the target fundamental TE-like cavity mode resonance wavelength, λ TE . Our design [29] has the following parameters: a nanobeam width w =0.58 λ TE , lattice constant (hole spacing) a =0.319 λ TE and elliptical hole minor radius r =0.087 λ TE . Furthermore, to minimize the scattering and maximize the cavity Q, the major radius of the elliptical hole array is decreased quadratically, over 30 periods, from r 1 =0.145 λ TE at the centre of the cavity, to r 30 =0.087 λ TE at its end. We modelled the devices using finite-difference time-domain methods, and found that they support both TM-like and TE-like resonances (with the fundamental TM-like resonance, λ TM , located at 0.9 λ TE ), with representative mode profiles shown in Fig. 3d,e , respectively. The dual mode nature of the triangular cross-section nanobeam cavities is of interest for applications in nonlinear optics and wavelength conversion [30] , [31] , [32] . Theoretical figures of merit for the fundamental cavity modes are Q-factors of Q TM ~1.3 × 10 5 and Q TE ~3.0 × 10 6 , with mode volumes V TM ~2.55( λ/n ) 3 and V TE ~2.26( λ/n ) 3 (the subscript again refers to the cavity mode transverse polarization). In addition, because of the gradual nature of the chirped lattice of air holes, the devices also support higher order longitudinal modes of both polarization. We note that devices shown in Fig. 3 are based on a design with fundamental cavity resonances located at λ TE =1,680-nm and λ TM =1,507-nm, respectively. Figure 3: High-Q diamond nanobeam photonic crystal cavities. SEM images of ( a ) diamond nanobeam photonic crystal cavities, with close-up ( b ) prospective and ( c ) top down views. Note, an ~35° etch angle was used to fabricate devices shown. Scale bars for SEM images in a – c correspond to 10, 1 and 2 μm, respectively. All SEM images were taken at a 60° stage tilt. Simulated cross-sectional and top down electric field intensity profiles of the fundamental quasi- ( d ) TE-like and ( e ) TM-like nanobeam photonic crystal cavity modes. Note, top down mode profiles correspond to top face of the nanobeam cavity. Theoretical figures of merit for the fundamental nanobeam photonic crystal cavity modes are Q-factors of Q TM ~1.3 × 10 5 and Q TE ~3.0 × 10 6 , with mode volumes V TM ~2.55 (λ/n) 3 and V TE ~2.26 (λ/n) 3 (the subscript refers to the cavity mode transverse polarization). ( f ) Representative normalized broadband spectrum of a fabricated diamond photonic crystal cavity collected by fibre taper measurement, with inset optical micrograph indicating the fibre taper coupling position. High-resolution spectra of the fundamental ( g ) TM-like and ( h ) TE-like cavity modes, with Lorentzian fits to the data also shown. The taper-loaded Q-factors (extracted from Lorentzian fits to the data) of the fundamental and second-order TM-like cavity modes were 24,000 and 3,700, respectively, while the first three TE-like cavity modes had loaded Q-factors of 183,000, 94,000 and 22,000, respectively. Full size image A normalized transmission spectrum of a representative diamond nanobeam cavity is shown in Fig. 3f . Two sets of transmission dips are observed, and are attributed to cavity resonances: dips located near 1,610-nm correspond to TE-like modes, while those located near 1,490-nm correspond to TM-like modes. The experimentally obtained fundamental resonance wavelengths for the two modes indicate λ TM,exp ~0.92 λ TE,exp , which is in good agreement with finite-difference time-domain predictions. The absolute values of cavity resonances are blue-shifted by roughly 5% from the target values, which is likely because of the uncertainty in the actual etch angle. The latter was previously estimated to deviate up to 2° degrees from the nominal value [33] (see Supplementary Discussion subsection (i) for cross-sectional analysis of fabrication diamond nanobeams). High-resolution spectra of fundamental TM-like and TE-like transverse cavity modes are shown in Fig. 3g,h , respectively. The loaded Q-factor of the fundamental TE-like cavity mode is remarkably high at Q TE ~ 183,000 and compares very well to the state-of-the-art silicon photonic crystal nanobeam cavities realized by standard fabrication techniques. We note that the loaded Q-factor of the fundamental TM-like nanobeam cavity is Q TM ~ 24,000. Nearly an order of magnitude reduction in cavity Q for this mode is likely due to its localization at the bottom apex of the nanobeam, which increases its losses by scattering from overlap with etched surfaces and leakage into the diamond substrate. Diamond optical nanocavities operating at visible wavelengths Finally, to utilize the broadband nature of diamond, we explored the potential of our angled-etching approach to realize optical cavities operating in visible and near-infrared. Visible diamond cavities are of great interest for the enhancement of emission properties of diamond’s luminescent defects, such as the negatively charged silicon vacancy centre (zero phonon line at λ ~737-nm) [34] , [35] , [36] and, in particular, the negatively charged nitrogen vacancy centre (NV − , with zero phonon line at λ ~637-nm and phonon side band up to nearly 800-nm) [37] , [38] , [39] . To realize visible band optical cavities in diamond, we scaled down all design parameters by a factor of ~2.5, and no additional modelling was needed. This design flexibility is an inherent property of angled-etching in which device thickness is coupled to its width. The same is not true for the planar technologies where one dimension is always fixed by the thickness of the device layer (for example, a 220-nm-thick silicon device layer in the case of silicon-on-insulator). Therefore, angled-etching allows for the integration of devices operating over a wide wavelength range (ultraviolet to mid-infrared) to be easily integrated on the same diamond chip. Figure 1c shows a fabricated visible band diamond racetrack resonators, with an ~500-nm-wide suspended waveguide and a 17.5-μm-bend radius. In such devices, the material segment supporting the free-standing waveguide is estimated to be ~90-nm thick. A broadband normalized transmission spectrum, shown in Fig. 4a , is obtained using a combination of tunable red laser (635–639-nm) and super-continuum source (see Methods for details). The insets of Fig. 4a display the fibre taper coupling position with the laser tuned off and on resonance; the diamond racetrack resonator lights up when the laser is resonant with the optical cavity. We note that because of the small coupling gap necessary at visible wavelengths, van der Waals attraction between the fibre taper and diamond device forced these measurements to be taken with the fibre taper touching the device. This ultimately limited coupling efficiency and measured cavity Q-factors. High-resolution spectra, collected with the tunable laser, of racetrack resonator cavity modes located at ~637-nm, are shown in Fig. 4b . The measured loaded Q-factors of the cavity modes were 33,000 and 59,000. For cavity modes at longer wavelengths, accurate measurement of their Q-factors by a tunable laser was not possible. However, Q-factors for resonances near 800-nm estimated from spectra collected by supercontinuum excitation exceed the resolution limit of the spectrometer, and thus were at least 10 4 . Therefore, free-standing diamond waveguides fabricated by angled-etching operate with low loss over a large, nearly 200-nm-wide bandwidth that covers visible and near-infrared wavelengths. 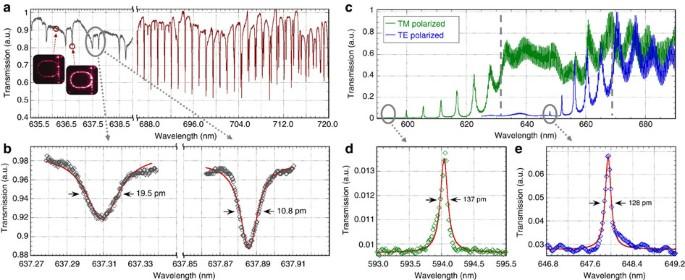Figure 4: Diamond optical nanocavities at visible wavelengths. (a) Normalized broadband transmission spectrum collected by fibre taper coupling from a diamond racetrack resonator (17.5-μm-bend radius and ~500-nm-beam width) using: (i) a tunable red laser and photodiode in 635–639-nm range (grey curve), and (ii) super-continuum source and spectrometer in 688–720-nm range (red curve). Two sets of supported resonances—the quasi-TE-like and TM-like waveguide modes—are again apparent. The insets reveal the fibre taper coupling position with a red laser tuned off and on resonance with the optical cavity. (b) Corresponding high-resolution spectra of two cavity modes near ~637-nm collected via a tunable laser, with Lorentzian fits to the data also shown. Lorentzian fits to each resonance inbyield loaded Q-factors of ~33,000 and 59,000. (c) Representative normalized broadband transmission spectra of a fabricated diamond nanobeam photonic crystal cavity operating in visible collected via free-space coupling at different input polarizations. High-resolution spectra of the fundamental (d) TM-like and (e) TE-like cavity modes, with Lorentzian fits to the data also shown. Lorentzian fits ind,eyield waveguide coupled Q-factors ofQTM~4,400 andQTE~5,100, respectively. Figure 4: Diamond optical nanocavities at visible wavelengths. ( a ) Normalized broadband transmission spectrum collected by fibre taper coupling from a diamond racetrack resonator (17.5-μm-bend radius and ~500-nm-beam width) using: (i) a tunable red laser and photodiode in 635–639-nm range (grey curve), and (ii) super-continuum source and spectrometer in 688–720-nm range (red curve). Two sets of supported resonances—the quasi-TE-like and TM-like waveguide modes—are again apparent. The insets reveal the fibre taper coupling position with a red laser tuned off and on resonance with the optical cavity. ( b ) Corresponding high-resolution spectra of two cavity modes near ~637-nm collected via a tunable laser, with Lorentzian fits to the data also shown. Lorentzian fits to each resonance in b yield loaded Q-factors of ~33,000 and 59,000. ( c ) Representative normalized broadband transmission spectra of a fabricated diamond nanobeam photonic crystal cavity operating in visible collected via free-space coupling at different input polarizations. High-resolution spectra of the fundamental ( d ) TM-like and ( e ) TE-like cavity modes, with Lorentzian fits to the data also shown. Lorentzian fits in d , e yield waveguide coupled Q-factors of Q TM ~4,400 and Q TE ~5,100, respectively. Full size image Figure 1d shows a representative diamond nanobeam cavity fabricated using the same design as previously described, with a target resonance for the fundamental TE-like cavity mode of λ TE =710-nm. In order to characterize such structures, a free-space coupling technique was used in lieu of fibre taper coupling, given the challenge of obtaining proper fibre alignment to small visible nanobeam cavities. The free-space measurement set-up (see Methods and Supplementary Fig. 5 ) allowed for in- and out-coupling of light at opposite ends of the nanobeam (using specifically placed notches as broadband couplers, see Supplementary Methods subsection (ii) for further description), thus enabling the free-space transmission measurements. A set of representative transmission spectra, collected via super-continuum excitation and spectrometer, taken from the same device but at different input/collection polarizations, are shown in Fig. 4c . These spectra correspond to TM-like (green curve) and TE-like (blue curve) polarized light transmitted through the diamond nanobeam waveguide that contains the optical cavity. Stop band (no transmission) and pass bands (high transmission) of the photonic crystal are clearly seen (the approximate location of the transition indicated with a dashed grey line), with the sharp resonances in the stop band corresponding to cavity modes. High-resolution spectra of the fundamental TM-like and TE-like cavity modes are shown in Fig. 4d,e , revealing waveguide coupled Q-factors of Q TM ~4,400 and Q TE ~5,100, respectively. Of the fabricated visible band nanobeam cavities, our best device had a measured Q-factor of Q TE ~8,200. In summary, high Q-factor racetrack and photonic crystal nanobeam cavities, realized using angled-etching nanofabrication scheme, have been demonstrated in bulk single-crystal diamond. Our devices feature Q-factors on par with those typically found in devices fabricated by conventional means, in standard photonic materials. Considering their wavelength scale mode volume ( V ~( λ/n ) 3 ), photonic crystal nanobeam cavities shown here feature the highest Q/V figure of merit demonstrated in single-crystal diamond to date. We have also showed that low loss waveguides carved from a bulk diamond crystal can be made using our novel tapered vertical support structures over a broad wavelength range. Our results demonstrate that single-crystal diamond is a viable nanophotonics platform, and will enable further breakthroughs in both classical and quantum optics. For instance, when fabricated around spectrally stable NV − or other colour centres [16] , [17] , [40] , diamond cavities will enable large enhancement of zero phonon line emission via the Purcell effect, as well as efficient collection of emitted photons. We emphasize that monolithic single-crystal diamond nanophotonic structures are ultimately compatible with post-processing techniques needed to stabilize implantation-defined colour centres, which often include high-temperature (~1,200 °C) annealing [41] . Moreover, high-Q optical nanocavities in diamond are an attractive nonlinear optics platform [18] and would combine the advantage of relatively large Kerr nonlinearity and large Raman gain, lack of two- or multiphoton absorption, and excellent thermal properties for the generation of on-chip high repetition rate frequency combs [18] , [42] and Raman lasers at exotic wavelenths [43] , [44] . The free-standing nature of angled-etched nanophotonic devices also offers mechanical degrees of freedom, allowing exploration of diamond optomechanics [45] , thus leveraging diamond’s unique mechanical and optical properties. Combining diamond optomechanical devices with NV − centres can result in on-chip hybrid quantum systems that rely on coherent spin-phonon–photon interactions for spin transduction and quantum state transfer [46] , [47] . Finally, our work will pave the way to realization of on-chip integrated photonic networks in other crystalline materials for which thin-film technology is not readily available. Angled-etching nanofabrication Standard optical grade, <100>-oriented, single-crystal diamond substrates (chemical vapour deposition grown, type IIa,<1-p.p.m. [N], Element Six) were polished to yield a surface roughness <5-nm root-mean-square (RMS) (performed by Delaware Diamond Knives). Received polished diamond substrates were then cleaned in a boiling mixture consisting of equal parts sulfuric acid, nitric acid and perchloric acid, followed by a pre-fabrication surface preparation [48] performed in a UNAXIS Shuttleline ICP-RIE. This included a 30-min etch with the following parameters: 400-W ICP power, 250-radio frequency (RF) power, 40-sccm Ar flow rate, 25-sccm Cl 2 flow rate and 8-mTorr chamber pressure, followed by a second 30-min etch with the following parameters: 700-W ICP power, 100-RF power, 50 sccm O 2 flow rate and 10-mTorr chamber pressure. The purpose of this pre-fabrication step was to reduce the surface roughness to <1-nm RMS and remove several microns from the top of the diamond substrate, which is likely strained due to initial mechanical polishing. Following surface preparation, a silica etch mask was patterned on the diamond substrates using hydrogen silsesquioxane (FOX-16 from Dow Corning)-negative resist and electron beam lithography. Exposed hydrogen silsesquioxane was developed in tetramethylammonium hydroxide (25% diluted solution). The silica etch mask pattern was transferred into the diamond via a conventional top down anisotropic plasma etch—also in the UNAXIS Shuttleline ICP-RIE—with the following parameters: 700-W ICP power, 100-RF power, 50-sccm O 2 flow rate, 2-sccm Cl 2 flow rate and 10-mTorr chamber pressure. The diamond was etched to a depth between 600- and 1,000-nm, depending on the particular device being fabricated. Following this, the angled-etching step was performed to realize the free-standing nanophotonic devices. Angled-etching was achieved using the same ICP-RIE parameters as the initial top down etch, but included housing the sample inside a specifically designed aluminium Faraday cage [20] to direct the plasma ions to the substrate surface at the intended angle (refer to Supplementary Methods subsection (i) for additional description). Two different Faraday cage designs were used (shown in Supplementary Fig. 1 and described in detail in Supplementary Methods subsection (i)), one of which was constructed to target a 45° etch angle, and the other for a target 60° etch angle. The resulting etch angles from these cage designs were measured to be ~35° and 50°, respectively. All diamond nanobeam cavities were fabricated at a 35° etch angle, while all diamond racetrack resonators were fabricated at a 50° etch angle. Following the oxygen-based plasma etching, the remaining etch mask was removed in concentrated hydrofluoric acid. Nanophotonic devices were cleaned in piranha solution before characterization. Fibre taper characterization at telecom and visible wavelengths Transmission measurements in the telecom band were collected via fibre taper coupling to suspended single-crystal diamond racetrack resonators. Fibre tapers were manufactured from SMF-28 fibre by the conventional flame anneal and pulling method [24] , resulting in a final diameter of ~1-μm. The fibre taper was mounted in a U-shaped configuration, resulting in self-tension of the taper region and allowing it to be positioned in close proximity to the desired diamond device. Since the diamond nanophotonic devices are raised above the diamond substrate in excess of 2 μm, dimpling the fibre taper was not necessary. The fibre taper was spliced into an optical set-up, and its position with respect to the device under test was precisely controlled via motorized stages with 50-nm encoder resolution. Two tunable lasers (Santec TSL-510, tuning range from 1,480- to 1,680-nm) were used, along with an inline fibre polarizer, and high gain InGaAs detector (EO Systems, IGA1.9-010-H) to record transmission spectra. All collected spectra were normalized by transmission data collected from an uncoupled position. For transmission measurements at visible wavelengths, fibre tapers were manufactured from commercial SM-600 fibre via wet etching in hydrofluoric acid [49] . Bare SM-600 fibre was again mounted in a U-shape configuration, followed by localized wet etching in hydrofluoric acid near the centre. The hydrofluoric acid was covered with a thin layer of o -xylene on top in order to promote gradual taper formation via the oil–water interface meniscus. A two-step etch process that included ~30-min of etching in concentrated hydrofluoric acid, followed by ~30- to 50-min etching in 5:1 buffered oxide etch, was used to thin the final taper region to a diameter of ~500–700-nm. Following visible fibre taper formation, the mounted fibre was again spliced into the same physical set-up as described for telecom band measurements. A fibre coupled super-continuum laser source (EXW-4, NKT Photonics) and optical spectrum analyser (OSA, HP 70950B, minimum resolution bandwidth of 0.08-nm) were used to collect broadband spectra in roughly the 680- to 800-nm band. To gauge the resolution of the OSA, a HeNe laser was connected directly to the OSA. Measurement of the resulting laser emission spectra yielded a line width ~70-pm, which is artificially broadened by the instrument resolution. As such, any measured Q-factor near and above 9,000 was deemed resolution-limited. To avoid this resolution limitation, a tunable red laser (New Focus Velocity TLB 6304 laser, coarse tuning range of 634.8–638.9-nm and fine tuning range of 70-pm) and visible band photodetector (New Focus 1801) were also used to collect transmission spectra. The fine tuning range of the laser was used to accurately measure the Q-factors of cavity modes supported by the diamond racetrack resonators within the ~4-nm coarse laser tuning range. Free-space transmission measurement at visible wavelengths Transmission measurements conducted by free-space coupling utilized a home-built confocal microscope in which a high numerical aperture (0.95) objective was used to focus laser light on the sample. The input laser optical path was scanned using a galvo mirror imaged on the back of the objective with a pair of lenses comprising a 4 f -imaging system. In addition, a beam splitter was placed between the input channel galvo mirror and the 4 f -imaging system in order to incorporate a collection channel with independent scanning control via its own set of galvo mirrors. The free-space coupling set-up was thus able to pump and collect light at two spatially separated positions, which allowed for free-space transmission measurements. Positioning of a target device under the objective was accomplished by precision-motorized stages. In order to couple light into and out of the diamond nanobeams, local broadband scatter centres in the form of notches—as seen in Fig. 1d of the main text—were incorporated at the two ends of fabricated nanobeam cavities. Light from a super-continuum laser source (EXW-4, NKT Photonics) was coupled into the diamond nanobeam cavity, with light out-coupled from the structure sent to a spectrometer. Free-space polarizers were also included in both the input and collection channels. A schematic of the free-space transmission measurement optical set-up is included as Supplementary Fig. 5 . How to cite this article: Burek, M. J. et al . High quality-factor optical nanocavities in bulk single-crystal diamond. Nat. Commun. 5:5718 doi: 10.1038/ncomms6718 (2014).